ILC2s and T cells cooperate to ensure maintenance of M2 macrophages for lung immunity against hookworms Defining the immune mechanisms underlying protective immunity to helminth infection remains an important challenge. Here we report that lung CD4 + T cells and Group 2 innate lymphoid cells (ILC2s) work in concert to block Nippostrongylus brasiliensis (Nb) development in the parenchyma within 48 h in mice. Immune-damaged larvae have a striking morphological defect that is dependent on the expansion of IL-13-producing ILC2 and CD4 + T cells, and the activation of M2 macrophages. This T-cell requirement can be bypassed by administration of IL-2 or IL-33, resulting in expansion of IL-13-producing ILC2s and larval killing. Depletion of ILC2s inhibits larval killing in IL-2-treated mice. Our results broaden understanding of ILC2’s role in immunity to helminths by demonstrating that they not only act as alarmin sensors, but can also be sustained by CD4 + T cells, ensuring both the prompt activation and the maintenance of IL-13-dependent M2 macrophage immunity in the lung. Despite many technological and chemotherapeutic advances, geohelminths continue to infect over a billion people worldwide [1] . Vaccination-induced protective immunity is seen as the most feasible solution for reducing these parasites’ significant morbidity and negative social impact on the developing world. A key evolutionary feature of the diverse intestinal parasites, including hookworms, Ascaris and Strongyloides, is that they include a migratory and a developmental stage in the lungs, before reaching the gut where they develop into adults [2] . The rodent parasite Nippostrongylus brasiliensis (Travassos, 1914) (Nb) models the salient features of helminth infection including skin penetration, migration from tissues to lung, maturation and egg production in the gut [3] . Primary infection stimulates host resistance to further reinfection through T helper type-2 (Th2)-mediated immune responses appearing in the skin, lung or gut [4] , [5] , [6] , [7] , [8] . Intriguingly, the Th2 effector mechanisms conferring resistance to Nb reinfection still remain to be fully characterized for the lung, which has been identified as a key site for priming acquired immunity against Nb [7] . An important associated feature of Nb infection is the significant damage to the epithelium and vasculature of the lung resulting from worm penetration and subsequent migration through the parenchyma into the airways [2] , [9] . In a primary infection, the host immune response to these events appears too slow to affect worm survival or fecundity. However, from 4 days after primary infection, enhanced anamnestic immune responses begin to develop that reduce the viability of worms and significantly reduce the lung haemorraging [10] . While several cell types have been described as participating in the repair mechanisms following Nb infection, their role in anamnestic immunity remains largely undefined. Alternatively activated macrophages [11] (M2) play a role in repairing the damage caused by Nb migration in the lung, both in the control of the initial haemorrhaging seen in the acute phase, and in the development of fibrosis and emphysema seen in the chronic phase [12] , as well as having a potential role in anamnestic immunity against Nb. Group 2 innate lymphoid cells (ILC2) have been shown to be critical for the interleukin (IL)-9-dependent repair of lungs damaged by Nb infection [13] . The role of ILC2s in protective immunity against helminths has been extensively studied with gut-associated ILC2s shown to promote the weep and sweep expulsion of helminths from the small intestine [14] , [15] ; however, the role of ILC2s in lung immunity against helminth infection, and more specifically their role in the potentiation of adaptive immunity, is unresolved. Here we investigate the lung cellular mechanisms that mediate immunity against reinfection by Nb in mice. We find that ILC2s acting in concert with CD4 + T cells and M2 macrophages in the lung parenchymal tissue play a crucial role in arresting Nb development and reducing worm burden in reinfected mice. Furthermore, we show that either IL-33- or IL-2-directed activation of ILC2s is sufficient to stimulate M2-mediated reduction of worm burden in the lungs, while in the context of naturally acquired immunity cooperation between ILC2s and CD4 + T cells is required for maintenance of anamnestic immunity. Naturally acquired protective immunity develops in the lung We sought to establish an experimental model to analyse the acquired immune response to Nb reinfection in the lungs of mice. When infectious stage 3 larvae (L3) are injected intravenously (i.v. ), the worms reach the lung within minutes, bypassing the skin and tissue phases to allow direct quantification of the numbers of worms that can be killed by lung-mediated immune processes ( Supplementary Fig. 1a ). The optimal time for lung-mediated killing of worms in i.v.-reinfected mice occurred between 9 and 30 days after reinfection, with a 60% reduction in worm viability ( Fig. 1a ). The number of worms that reached the lungs was reduced by a further 20% if reinfection occurred by the subcutaneous (s.c.) route ( Fig. 1a,b , Supplementary Fig. 1b ). We therefore focused our studies of anamnestic immunity on the lung, using the i.v. larvae administration model with a time interval of 30 days between primary infection and reinfection. 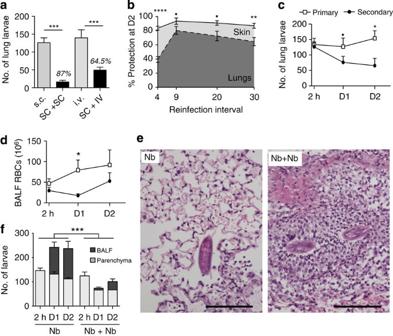Figure 1: The lung is a key site of immunity toN. brasiliensisreinfection. (a) Mice were primed by s.c. infection and reinfected 30 days later by either s.c. or i.v. inoculation (dark grey). Naïve mice were infected by either s.c.- or i.v. inoculation (light grey). Lung worm burden was assessed 2 days after challenge. The calculated percentage of protection is indicated on the graph (n=5 mice, mean+s.e.m., representative of three independent experiments, ANOVA). (b) Mice were s.c. infected 4, 9, 20 or 30 days before i.v.- or s.c. reinfection. Lung worm burden was assessed 2 days after challenge and protection was calculated as a percentage (n=5 mice, mean+s.e.m., representative of two independent experiments, ANOVA). (c,d) Number ofN. brasiliensislarvae in lung tissue (c) and number of red blood cells in the BALF (d) 2, 24 or 48 h post-primary (open boxes) or secondary (closed circles) i.v. infection (with 30 days between primary and reinfection;n=5 mice, mean+s.e.m., representative of two independent experiments, ANOVA). (e) Haematoxylin and eosin staining of lung sections at 48 h post-primary (Nb) or i.v. reinfection (Nb+Nb) infection. Scale bar, 100 μm. (f) Number ofN. brasiliensislarvae in the lung parenchyma (light grey bars) or airway space, measured in BALF (dark grey bars), 2, 24 or 48 h post-primary or i.v. reinfection (n=5 mice, mean+s.e.m., representative of two independent experiments, ANOVA). NS, non-significant;P>0.05;▪P<0.07; *P<0.05; **P<0.01; ***P<0.001; ****P<0.0001. Figure 1: The lung is a key site of immunity to N. brasiliensis reinfection. ( a ) Mice were primed by s.c. infection and reinfected 30 days later by either s.c. or i.v. inoculation (dark grey). Naïve mice were infected by either s.c.- or i.v. inoculation (light grey). Lung worm burden was assessed 2 days after challenge. The calculated percentage of protection is indicated on the graph ( n =5 mice, mean+s.e.m., representative of three independent experiments, ANOVA). ( b ) Mice were s.c. infected 4, 9, 20 or 30 days before i.v.- or s.c. reinfection. Lung worm burden was assessed 2 days after challenge and protection was calculated as a percentage ( n =5 mice, mean+s.e.m., representative of two independent experiments, ANOVA). ( c , d ) Number of N. brasiliensis larvae in lung tissue ( c ) and number of red blood cells in the BALF ( d ) 2, 24 or 48 h post-primary (open boxes) or secondary (closed circles) i.v. infection (with 30 days between primary and reinfection; n =5 mice, mean+s.e.m., representative of two independent experiments, ANOVA). ( e ) Haematoxylin and eosin staining of lung sections at 48 h post-primary (Nb) or i.v. reinfection (Nb+Nb) infection. Scale bar, 100 μm. ( f ) Number of N. brasiliensis larvae in the lung parenchyma (light grey bars) or airway space, measured in BALF (dark grey bars), 2, 24 or 48 h post-primary or i.v. reinfection ( n =5 mice, mean+s.e.m., representative of two independent experiments, ANOVA). NS, non-significant; P >0.05; ▪ P <0.07; * P <0.05; ** P <0.01; *** P <0.001; **** P <0.0001. Full size image To determine the location and timing of immune-mediated killing of Nb larvae, we tracked larvae fate in the lungs of i.v.-reinfected mice. Two hours post i.v. infection, the number of viable larvae recovered from reinfected mice was unaffected ( Fig. 1c ). However, at both 24 and 48 h post i.v. infection, a significant reduction in the number of worms in the lung was observed in reinfected mice ( Fig. 1c ), with no larvae found in the gut or stomach, confirming that the larvae were killed in the lungs ( Supplementary Fig. 1c ). We noted that the decrease in Nb numbers in the lungs of reinfected mice correlated with a decrease in erythrocytes in the bronchoalveolar lavage fluid (BALF, Fig. 1d ), possibly attributable to both a reduction in Nb-induced haemorrhaging and accelerated lung repair mechanisms, rather than to reduced numbers of worms reaching the lung as reported previously [5] , [12] . Histological analysis of the lungs of reinfected mice revealed the appearance at 48 h of intense inflammatory foci around trapped larvae, characterized by epithelial lung bronchi hyperplasia, with focally moderate neutrophilic infiltrate and scattered histiocytes. This was in contrast to the histology seen in the lungs of mice 48 h after a primary i.v. infection, with oblique sections of worm being quite visible at 48 h, but with little evidence of inflammatory cell aggregation, thus suggesting an active in situ trapping and killing of the worms during i.v. reinfection ( Fig. 1e ). To exclude the possibility that the reduced numbers of worms in reinfected mice merely reflected clearance and passage to the gut due to increased exudate flow, we followed in detail the numbers of larvae at each stage of the migratory route, including lung parenchyma, airways, stomach and small intestine in both i.v.-infected naïve or previously infected mice. Two hours after i.v. infection, worm counts in lung parenchyma were identical in both primary and reinfected lungs, with no worms having migrated to the airways ( Fig. 1f ). However, by 24 and 48 h post i.v. infection, the majority of worms reaching the lungs of a naïve mouse had started to migrate through the airways, eventually appearing in the stomach and small intestine ( Fig. 1f , Supplementary Fig. 1c ). In contrast, the numbers of worms reaching the airways were reduced in i.v.-reinfected mice, with little to no worms being detected in the stomach or small intestine at any time after infection ( Fig. 1f , Supplementary Fig. 1c ). These observations, and our findings that i.v.-injected dead worms and latex beads introduced to the lungs of naïve mice could not be detected in the airways ( Supplementary Fig. 1d ), rule out the possibility that the reduction in worm numbers is simply due to enhanced exudatory clearance mechanisms, instead suggesting direct killing of L3 in the parenchyma. Lung immunity leads to a fatal worm defect during molt 3 We compared the morphology and developmental features of worms recovered from the lungs of naïve mice with the worms that could be isolated from lungs of reinfected mice. Larvae isolated from the lung parenchyma of infected naïve mice presented with molt 3 (developing from L3 to L4) early-differentiation characteristics including appearance of dark pigmented intestinal granules, while larvae harvested from airways had an advanced molt 3 morphology, with observable stage 4 cephalic expansion, fully developed and pigmented intestine and the beginning of sex differentiation [16] ( Supplementary Fig. 2a ). In contrast, larvae harvested from the lung parenchyma of i.v.-reinfected mice have a strikingly different appearance, with 45% of the larvae presenting a morphological defect, in which the feeding apparatus has protruded through the excretory–secretory pore (hereafter referred to as immune-related excretory protrusion defect or IREP) ( Fig. 2a,b , Supplementary Fig. 2b ). This IREP was also observed in worms isolated from lungs of primary infected mice, albeit with a much lower incidence averaging at 15%, and may be one of the causes of the natural attrition during the parasite life cycle ( Fig. 2b ). Associated with the marked increase in IREP defects seen in worms from the lungs of i.v.-reinfected mice, we observed a moulting defect, as shown by reduction of several morphological larval features that are known to increase during the moulting process [16] , including a reduction in the total length of larvae ( Supplementary Fig. 2c ), a reduction in the length of the oesophagus ( Supplementary Fig. 2d ), and a less pronounced intestinal pigmentation ( Supplementary Fig. 2e ). Finally, using intrinsic ATP activity as a surrogate for worm fitness, we noted that larvae isolated from the lungs of i.v.-reinfected mice had significantly reduced fitness compared with primary infected mice ( Fig. 2c ). Of note was the observation that larvae isolated from i.v.-reinfected mice were intimately associated with immune cells, such as macrophages, eosinophils and neutrophils ( Fig. 2d ). No such cell attachment has been observed on larvae harvested from primary i.v.-infected mice. We conclude that the immune response to Nb reinfection confers protection to the host by compromising Nb viability at the moulting stage and by significantly limiting the passage of L3 from the lung parenchyma into the airways. 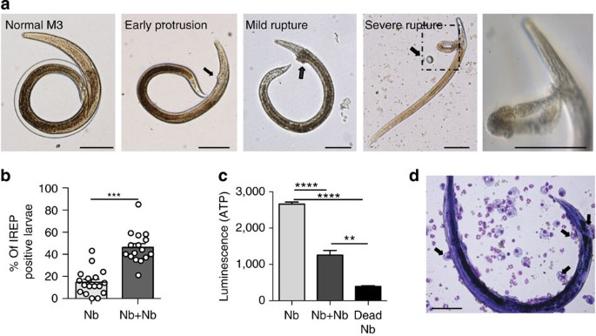Figure 2: Larval developmental arrest occurs in the lungs of Nb-reinfected mice. (a) Bright-field microscopy showing increasing severity of larval developmental defects from normal larvae at the moult 3 stage (M3) obtained by migration at 37 °C, to protrusion of the intestine. The larvae obtained by liberase digestion presented similar features, with more immune cells attached. Last panel shows the IREP defect in more detail. Scale bars, 100 μm. (b) Percentage of larvae displaying the IREP defect in the lungs of mice 2 days post-primary (Nb) or secondary (Nb+Nb) i.v. infection. Each dot represents an individual mouse in which 20–40 larvae were studied (n=2–3 mice, mean+s.e.m., pooled from six independent experiments,t-test). (c) ATP measurement of pooled larvae harvested from the lungs of mice infected once or twice, compared with a control group of larvae killed by boiling (n=13, mean+s.e.m., ANOVA) (d) Giemsa-stained cytospin of larva from liberase-digested lung tissue at day 2 post secondary infection, surrounded and adhered to by macrophages and eosinophils. Scale bar, 50 μm. **P<0.01; ***P<0.001; ****P<0.0001. Figure 2: Larval developmental arrest occurs in the lungs of Nb-reinfected mice. ( a ) Bright-field microscopy showing increasing severity of larval developmental defects from normal larvae at the moult 3 stage (M3) obtained by migration at 37 °C, to protrusion of the intestine. The larvae obtained by liberase digestion presented similar features, with more immune cells attached. Last panel shows the IREP defect in more detail. Scale bars, 100 μm. ( b ) Percentage of larvae displaying the IREP defect in the lungs of mice 2 days post-primary (Nb) or secondary (Nb+Nb) i.v. infection. Each dot represents an individual mouse in which 20–40 larvae were studied ( n =2–3 mice, mean+s.e.m., pooled from six independent experiments, t -test). ( c ) ATP measurement of pooled larvae harvested from the lungs of mice infected once or twice, compared with a control group of larvae killed by boiling ( n =13, mean+s.e.m., ANOVA) ( d ) Giemsa-stained cytospin of larva from liberase-digested lung tissue at day 2 post secondary infection, surrounded and adhered to by macrophages and eosinophils. Scale bar, 50 μm. ** P <0.01; *** P <0.001; **** P <0.0001. Full size image Neutrophil depletion compromises skin-mediated protection Neutrophils have been associated with lung haemorrhagic foci in Nb-infected mice [12] , [17] and recently have been shown to be important for the priming of an anamnestic protective immune response against Nb [18] . Furthermore, neutrophil-dependent extracellular traps have been shown to compromise Strongyloides venezuelensis larval migration in skin [19] . Collectively, these reports and our detection of neutrophils in lung inflammatory foci surrounding larvae in reinfected mice suggested neutrophils may be involved in the immune-mediated reduction in worm burden in the lungs of reinfected mice. We found that the depletion of neutrophils before reinfection with Nb had no effect on the immune-mediated decrease in viable worm numbers in the lung indicating that neutrophils are not required for lung protection against Nb ( Fig. 3a , Supplementary Fig. 3a,b ). Similarly, depletion of neutrophils during the primary Nb infection had no effect on subsequent immunity against migrating lung larvae seen during reinfection. However, we did observe a significant abrogation of skin-mediated protection following neutrophil depletion, with fewer larvae found trapped in the skin and more larvae able to be recovered from the lungs ( Fig. 3b,c ). 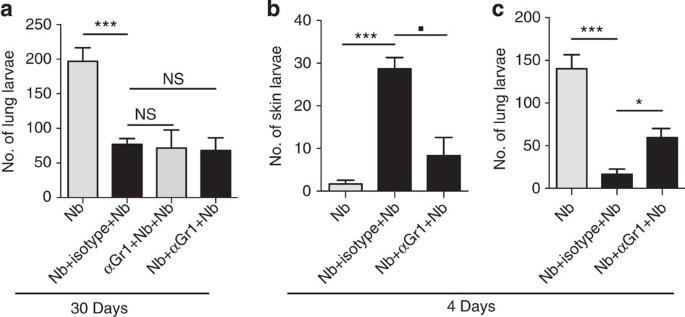Figure 3: Neutrophils are required for immunity against Nb larvae in the skin, but not in the lung. (a) Number ofN. brasiliensislarvae in the lungs 2 days post-primary (Nb) or i.v. reinfection (Nb+Nb; reinfection infection occurs 30 days after primary infection). Neutrophils were depleted in the relevant groups with 250 μg anti-Gr1 antibody (RB6–8C5) 1 day before priming (αGr1+Nb+Nb) or one day before i.v. reinfection (Nb+αGr1+Nb;n=5 mice, mean+s.e.m., representative of two independent experiments, ANOVA). (b,c) Number ofN. brasiliensislarvae in the skin (b) and lungs (c) 2 days post-s.c. primary infection or reinfection (reinfection infection occurs 4 days after primary infection). Neutrophils were depleted in the relevant groups 1 day before s.c. reinfection (n=5 mice, mean+s.e.m., representative of two independent experiments, ANOVA). NS, non-significant;▪P<0.07; *P<0.05; ***P<0.001. Figure 3: Neutrophils are required for immunity against Nb larvae in the skin, but not in the lung. ( a ) Number of N. brasiliensis larvae in the lungs 2 days post-primary (Nb) or i.v. reinfection (Nb+Nb; reinfection infection occurs 30 days after primary infection). Neutrophils were depleted in the relevant groups with 250 μg anti-Gr1 antibody (RB6–8C5) 1 day before priming (αGr1+Nb+Nb) or one day before i.v. reinfection (Nb+αGr1+Nb; n =5 mice, mean+s.e.m., representative of two independent experiments, ANOVA). ( b , c ) Number of N. brasiliensis larvae in the skin ( b ) and lungs ( c ) 2 days post-s.c. primary infection or reinfection (reinfection infection occurs 4 days after primary infection). Neutrophils were depleted in the relevant groups 1 day before s.c. reinfection ( n =5 mice, mean+s.e.m., representative of two independent experiments, ANOVA). NS, non-significant; ▪ P <0.07; * P <0.05; *** P <0.001. Full size image CD4 + T cell and ILC2 cytokine responses mediate Nb killing To identify the lung immune cell types and cytokines mediating the worm developmental defects in i.v.-reinfected mice, we investigated the effect of host STAT6 −/− deficiency on worm viability. Stat6 −/− mice failed to reduce worm numbers in the lung when i.v. reinfected as compared with wild-type C57BL/6 (B6) mice ( Fig. 4a ). Furthermore, the skewed distribution of larvae to the lung parenchyma seen in i.v.-reinfected B6 mice was not observed in Stat6 −/− mice, indicating a role for STAT6 signalling, and potentially the role of IL-4 and IL-13 production, in host responses that prevent larvae from developing and migrating from the lung parenchyma to the airways ( Fig. 4a ). Also the morphology of larvae isolated from Stat6 −/− lung parenchyma was identical in both primary and secondary infection (14.8%±5.3 IREP in reinfected Stat6 −/− mice versus 8.5%±3.6 in primary infected Stat6 −/− ). Interestingly, we observed that the IL-4-deficient mice ( Fig. 4b ) and anti-IL-13-treated mice ( Fig. 4c ) maintained immunity to i.v. reinfection with only a few larvae being recoverable from the airways. However, treatment of IL-4-deficient mice with anti-IL-13 antibody abrogated all lung immunity to reinfection, indicating redundancy in IL-4 and IL-13 production during lung-mediated immunity, which is distinct from the recently described role for IL-4 in skin immunity to Nb [5] . 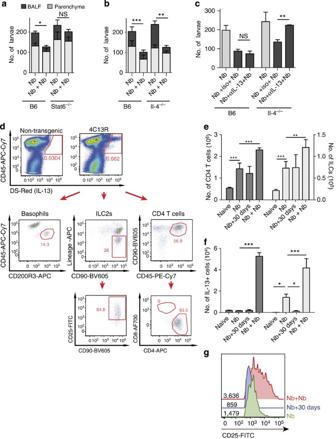Figure 4: Lung immunity towardsN. brasiliensisreinfection is dependent on IL-13-producing T cells and ILC2s. (a,b) Number ofN. brasiliensislarvae in the airways, measured in BALF (dark grey) or lung parenchyma (light grey) of Stat6−/−(a), Il-4−/−(b) or wild-type (B6) mice 2 days post-primary (Nb) or (Nb+Nb) i.v. reinfection (n=5 mice, mean+s.e.m., representative of two independent experiments, ANOVA on total larvae number). (c) Number of lung larvae 2 days post infection in C56Bl/6 or Il-4−/−mice treated for 1 week of IL-13 blockade before i.v. reinfection or with matched isotype control antibody (AbbVie,n=4 mice, mean+s.e.m., ANOVA). (d) Representative flow cytometry plots of IL-13+cells in i.v.-reinfected–infected wild-type and 4C13R transgenic mice. All cell types are identified as live and DS-Red+. Basophils are further identified by expression of CD200R3 and CD45mid. ILC2s are identified as lineage negative CD90+CD25+. CD4+T cells are identified as CD90+CD4+. (e) Number of CD4+T cells (dark grey bars) and ILC2s (light grey bars) in the lung tissue of naïve 4C13R mice, at days 2 after i.v. primary infection (Nb) and 30 post-primary s.c. infection (Nb+30 days) and at 2 days after i.v. reinfection (Nb+Nb,n=5, mean+s.e.m., representative of two independent experiments, ANOVA). (f) Number of IL-13+CD4+T cells and ILC2s as identified ind(n=5, mean+s.e.m., representative of two independent experiments, ANOVA). (g) Histogram of CD25 expression on ILC2s identified ind. NS, non-significant;P>0.05; *P<0.05; **P<0.01; ***P<0.001. Figure 4: Lung immunity towards N. brasiliensis reinfection is dependent on IL-13-producing T cells and ILC2s. ( a , b ) Number of N. brasiliensis larvae in the airways, measured in BALF (dark grey) or lung parenchyma (light grey) of Stat6 −/− ( a ), Il-4 −/− ( b ) or wild-type (B6) mice 2 days post-primary (Nb) or (Nb+Nb) i.v. reinfection ( n =5 mice, mean+s.e.m., representative of two independent experiments, ANOVA on total larvae number). ( c ) Number of lung larvae 2 days post infection in C56Bl/6 or Il-4 −/− mice treated for 1 week of IL-13 blockade before i.v. reinfection or with matched isotype control antibody (AbbVie, n =4 mice, mean+s.e.m., ANOVA). ( d ) Representative flow cytometry plots of IL-13 + cells in i.v.-reinfected–infected wild-type and 4C13R transgenic mice. All cell types are identified as live and DS-Red + . Basophils are further identified by expression of CD200R3 and CD45 mid . ILC2s are identified as lineage negative CD90 + CD25 + . CD4 + T cells are identified as CD90 + CD4 + . ( e ) Number of CD4 + T cells (dark grey bars) and ILC2s (light grey bars) in the lung tissue of naïve 4C13R mice, at days 2 after i.v. primary infection (Nb) and 30 post-primary s.c. infection (Nb+30 days) and at 2 days after i.v. reinfection (Nb+Nb, n =5, mean+s.e.m., representative of two independent experiments, ANOVA). ( f ) Number of IL-13 + CD4 + T cells and ILC2s as identified in d ( n =5, mean+s.e.m., representative of two independent experiments, ANOVA). ( g ) Histogram of CD25 expression on ILC2s identified in d . NS, non-significant; P >0.05; * P <0.05; ** P <0.01; *** P <0.001. Full size image To determine the major cell types producing IL-13 during the first 2 days of the immune response to Nb i.v. reinfection, we utilized the IL-4/IL-13 dual reporter mice 4C13R [20] , [21] ( Fig. 4d ). As previously reported, CD4 + T cells, basophils, neutrophils and eosinophils were the main IL-4 producing cells [7] , [22] and ILC2s, CD4 + T cells, and basophils were the major IL-13-producing cells that could be detected during the lung immune response to Nb ( Fig. 4d , Supplementary Fig. 4a ). The role of basophil-derived IL-13 and IL-4 in the lung-protective response was precluded by the observation that IL-3-deficient mice were fully immune to Nb reinfection in the lung, as basophil responses in Nb infection are IL-3 dependent [23] ( Supplementary Fig. 4b ). Similarly, eosinophils have been found to play no role in lung-mediated immunity to Nb [7] . We were intrigued by the relatively high numbers of IL-13-producing ILC2s appearing in the lung and thus examined their potential role in the context of immunity to reinfection with Nb. We therefore followed ILC2 numbers and cytokine expression from the lungs of either naïve, 2 days post primary, 30 days post primary, 2 days post reinfected mice, as compared with CD4 + T-cell responses. We observed a two–threefold elevation in numbers of IL-13-producing CD4 + T cells and ILC2s that was maintained for at least 30 days following primary infection ( Fig. 4e,f ). When challenged with i.v. reinfection, the number of CD4 + T cells and ILC2 increased to significantly higher levels than seen in the primary response. Of note was that the increased number of IL-13-producing ILC2s was also accompanied by a significant upregulation in CD25 marker expression indicating a potential pathway for regulation of ILC2s by the CD4 + T-cell-derived cytokine IL-2 ( Fig. 4g ). Cytokine-activated ILC2s reduce worm viability in the lung The preceding data implicate ILC2s as a strong candidate cell population for mediating the larval immune killing seen during reinfection. Supporting this view is their location in the lung parenchyma ( Supplementary Fig. 5 ) and the reported observation that ILC2s can be activated by IL-2 or IL-33 (refs 20 , 24 , 25 , 26 ). How the ILC2s might be alerted to the presence of tissue migrating larvae remains a key issue. The alarmin IL-33 has been shown to be released by lung epithelial cells during Nb infection, and it has been demonstrated to be important in regulating the subsequent response to tissue damage following Nb infection, as well as being required for ILC2s expansion during reinfection [24] , [26] , [27] . We investigated whether IL-33-mediated activation of ILCs was sufficient for killing worms in the lung by using a model of intranasal administration of recombinant murine IL-33 (rmIL-33) before Nb infection ( Fig. 5a ). Four days after rmIL-33 intranasal administration, there was a concomitant significant decrease in the numbers of lung Nb larvae compared with control infected mice, along with a significant increase in the numbers of ILC2s ( Fig. 5b ). The decrease in worm viability in the lungs was also observed in Rag1 −/− mice indicating that the IL-33-induced killing could occur independently of CD4 + T cells in this model ( Fig. 5c ). 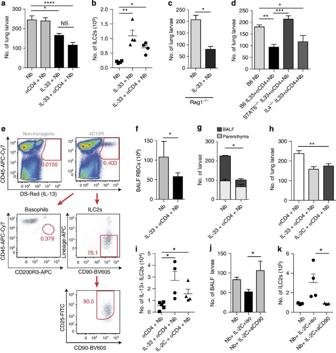Figure 5: IL-33- or IL-2-induced ILC2s can mediate lung immunity to NB infection. (a,b) Mice were treated intranasally with rmIL-33 or PBS and/or intraperitoneally with anti-CD4 (GK1.5) antibody, 2 days before i.v. infection with Nb. Lungs were harvested 2 days after infection (n=4 mice, mean+s.e.m., pool of four independent experiments, ANOVA). (a) Number ofN. brasiliensislarvae in the lung 2 days post-primary infection (Nb), and with anti-CD4 and/or intranasal rmIL-33 or PBS treatment. (b) Number of ILC2s in the lung after primaryN. brasiliensisinfection (Nb), and after intranasal rmIL-33 or PBS administration, in the presence or absence of anti-CD4. (c) Number ofN. brasiliensislarvae in the lung of Rag1−/−mice 2 days post i.v. primary infection following intranasal rmIL-33 or PBS treatment (n=5, mean+s.e.m., representative of two independent experiments,t-test). (d) Number ofN. brasiliensislarvae in the lung 2 days post-primary infection (Nb) in wild-type B6, Stat6−/−and Il-4−/−mice (n=5 mice, mean+s.e.m., representative of two independent experiments, ANOVA) after rmIL-33 and anti-CD4 administration. (e) Representative flow cytometry analysis of IL-13+cells using the 4C13R reporter mice, treated as ina. (f) Number of red blood cells in the BALF of mice treated as ina, (n=4 mice, mean+s.e.m., representative of two independent experiments,t-test). (g) Differential larvae number in the airways (dark grey bars) or lung parenchyma (light grey bars,n=4 mice, mean+s.e.m., representative of two independent experiments,t-test). (h) Number ofN. brasiliensislarvae in the lung, 2 days post-primary i.v. infection with anti-CD4 administration and either intranasal rmIL-33 or intraperitoneal IL-2C treatment (n=4 mice, mean+s.e.m., pool of two independent experiments, ANOVA). (i) Number of IL-13+ILC2s in the lung, 2 days post-primary infection with anti-CD4 administration and either intranasal rmIL-33 or intraperitoneal IL-2C treatment (n=5, mean+s.e.m., ANOVA). (j) Number ofN. brasiliensislarvae in the BALF, 2 days post-primary infection and intraperitoneal IL-2C or PBS treatment of Rag1−/−,treated daily with anti-CD90 or isotype control (30H12,n=4 mice, mean+s.e.m., ANOVA). (k) Number of ILC2s in the lung, 2 days post primary infection and intraperitoneal IL-2C treatment of Rag1−/−, treated daily with anti-CD90 or isotype control (n=3–5, mean+s.e.m., ANOVA). *P<0.05; **P<0.01; ***P<0.001; ****P<0.0001. RBC, red blood cell. Figure 5: IL-33- or IL-2-induced ILC2s can mediate lung immunity to NB infection. ( a , b ) Mice were treated intranasally with rmIL-33 or PBS and/or intraperitoneally with anti-CD4 (GK1.5) antibody, 2 days before i.v. infection with Nb. Lungs were harvested 2 days after infection ( n =4 mice, mean+s.e.m., pool of four independent experiments, ANOVA). ( a ) Number of N. brasiliensis larvae in the lung 2 days post-primary infection (Nb), and with anti-CD4 and/or intranasal rmIL-33 or PBS treatment. ( b ) Number of ILC2s in the lung after primary N. brasiliensis infection (Nb), and after intranasal rmIL-33 or PBS administration, in the presence or absence of anti-CD4. ( c ) Number of N. brasiliensis larvae in the lung of Rag1 −/− mice 2 days post i.v. primary infection following intranasal rmIL-33 or PBS treatment ( n =5, mean+s.e.m., representative of two independent experiments, t -test). ( d ) Number of N. brasiliensis larvae in the lung 2 days post-primary infection (Nb) in wild-type B6, Stat6 −/− and Il-4 −/− mice ( n =5 mice, mean+s.e.m., representative of two independent experiments, ANOVA) after rmIL-33 and anti-CD4 administration. ( e ) Representative flow cytometry analysis of IL-13 + cells using the 4C13R reporter mice, treated as in a . ( f ) Number of red blood cells in the BALF of mice treated as in a , ( n =4 mice, mean+s.e.m., representative of two independent experiments, t -test). ( g ) Differential larvae number in the airways (dark grey bars) or lung parenchyma (light grey bars, n =4 mice, mean+s.e.m., representative of two independent experiments, t -test). ( h ) Number of N. brasiliensis larvae in the lung, 2 days post-primary i.v. infection with anti-CD4 administration and either intranasal rmIL-33 or intraperitoneal IL-2C treatment ( n =4 mice, mean+s.e.m., pool of two independent experiments, ANOVA). ( i ) Number of IL-13 + ILC2s in the lung, 2 days post-primary infection with anti-CD4 administration and either intranasal rmIL-33 or intraperitoneal IL-2C treatment ( n =5, mean+s.e.m., ANOVA). ( j ) Number of N. brasiliensis larvae in the BALF, 2 days post-primary infection and intraperitoneal IL-2C or PBS treatment of Rag1 −/−, treated daily with anti-CD90 or isotype control (30H12, n =4 mice, mean+s.e.m., ANOVA). ( k ) Number of ILC2s in the lung, 2 days post primary infection and intraperitoneal IL-2C treatment of Rag1 −/− , treated daily with anti-CD90 or isotype control ( n =3–5, mean+s.e.m., ANOVA). * P <0.05; ** P <0.01; *** P <0.001; **** P <0.0001. RBC, red blood cell. Full size image We next wanted to confirm whether ILC2s were mediating their effects on Nb in the lung via the expression of IL-13 such as has been reported for ILC2s mediating gut helminth expulsion [15] . We found that IL-33-induced worm killing was abrogated in Stat6 −/− mice, but was maintained in Il-4 −/− , indicating that the killing effect occurred at least partially via an IL-13-dependent mechanism, as seen in natural resistance to i.v. reinfection ( Fig. 5d ). We further confirmed that ILC2s were the main source of IL-13 in the lung using intranasal rmIL-33 administration in CD4-depleted 4C13R reporter mice ( Fig. 5e ). Administration of rmIL-33 was also associated with a reduction in the degree of lung haemorrhaging to levels equivalent to those seen in i.v.-reinfected B6 mice ( Fig. 5f ). Moreover, the number of larvae that reached the airways was reduced in mice that received rmIL-33 treatment before infection ( Fig. 5g ), suggesting that the IL-33-induced ILC2 response results in a reduction in worm survival similar to the one seen in natural resistance to reinfection. Indeed, the IREP phenotype was more prevalent in rmIL-33 treated mice, as compared with controls (14.4%±3.6 IREP in IL-33-treated mice versus 3.1%±1.3 in untreated mice as a frequency of total lung worm number). To further confirm the role of ILC2s in the lung worm killing, we used exogenous administration of IL-2-anti-IL-2-immune-complexes (IL-2C) as an alternate pathway for inducing ILC2 expansion and activation [20] , [25] . Similar to rmIL-33 administration, systemic IL-2C treatment resulted in decreased worm recovery from the lung of Nb i.v.-infected mice and concomitant increased numbers of IL-13-producing ILC2s ( Fig. 5h–k ). Importantly, the expansion of ILC2s and the associated larval killing in Rag1 −/− mice treated with IL-2C was abrogated by in vivo depletion with anti-CD90 antibody indicating a role for ILC2s in protection ( Fig. 5j,k ). Taken together, these results indicate the potential role of IL-13-producing ILC2s in mediating protective immunity against Nb albeit under the tight regulation by the cytokines IL-33 or IL-2 resulting from tissue damage or CD4 + T-cell activation, respectively. ILC2-mediated immunity against Nb requires CD4 + T cells Priming of CD4 + T cells has been shown to be required for the development of lung immunity to Nb reinfection [6] , [7] ; however, the potential for these and other immune cell types in mediating the effector responses against Nb larvae remains undetermined. In particular, the elevated numbers of IL-13-producing ILC2s seen in the lungs of mice 30 days post primary infection suggested that these cells could play a role in the rapid secondary immune response that reduces viability of migrating lung larvae ( Fig. 4e,f ). CD4 + T cells were proven to be sufficient to mediate protection as adoptive transfer of activated CD4 + T cells from previously infected mice conferred protection to Nb in recipient mice ( Fig. 6a ). We next investigated whether CD4 + T cells mediated their activity directly as effector cells or whether they worked indirectly through the regulation of other cytokine-producing populations such as the ILC2s. To address this, we depleted CD4 + T cells from Nb immune mice either 1 or 7 days before i.v. reinfection. Strikingly, depletion of CD4 + T cells 1 day before i.v. reinfection did not interfere with the reduction of worm numbers in the lung, suggesting that CD4 + T cells do not directly mediate natural resistance to reinfection ( Fig. 6b ). However, depletion of CD4 + T cells 7 days before i.v. reinfection abrogated the immune-mediated killing of Nb in the lung ( Fig. 6b ) with an associated reappearance of haemorrhaging to the level seen in primary infections ( Fig. 6c ). 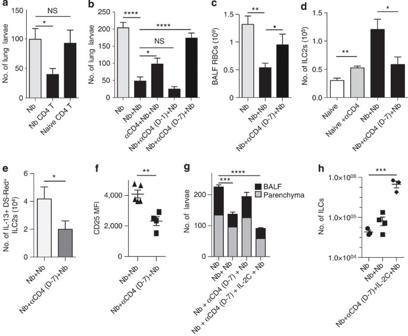Figure 6: CD4+T cells are required for the maintenance of ILC2-induced immunity toN. brasiliensis. (a) Number ofN. brasiliensislarvae in the lung 2 days post primary infection (Nb), or after intranasal adoptive transfer of CD4+T cells isolated from naïve mice or mice infected 29 days before transfer (n=5 mice, mean+s.e.m., representative of two independent experiments, ANOVA). (b) Number ofN. brasiliensislarvae in the lungs of mice 2 days post primary infection (Nb) and i.v. reinfection (Nb+Nb), or after CD4+T-cell depletion before primary infection (αCD4+Nb+Nb), and 7 days or 24 h before secondary infection (Nb+αCD4+Nb;n=5 mice, mean+s.e.m., representative of two independent experiments, ANOVA). (c) Number of red blood cells in the BALF of mice given a primary (Nb) or secondary (Nb+Nb) infection, and after CD4+T-cell depletion 7 days before the secondary (Nb+αCD4+Nb). (d) Number of ILC2s in the lung of naïve mice or mice 2 days post secondary infection, with or without CD4+depletion one week before reinfection (n=3–5, mean+s.e.m., representative of three independent experiments, ANOVA). (e) Number of IL-13+ILC2s in the lung 2 days post challenge infection or with CD4+depletion one week before reinfection (n=5, mean+s.e.m., representative of two independent experiments,t-test). (f) Mean fluorescent intensity of CD25 expression on lung ILC2s, as ine. (g) Differential larvae number in the airways and lung parenchyma of mice with primary (Nb) or i.v. reinfection (Nb+Nb), after CD4 depletion and/or intraperitoneal IL-2C treatment for 7 days before challenge (n=5, mean+s.e.m., representative of two independent experiments, ANOVA). (h) Number of ILC2s in the lungs of i.v.-primary infected (Nb) or reinfected (Nb+Nb) mice, and with CD4 depletion and IL-2C treatment for 7 days before challenge (n=5, mean+s.e.m., ANOVA). NS, non-significant;P>0.05;▪P<0.07; *P<0.05; **P<0.01; ***P<0.001; ****P<0.0001. Figure 6: CD4 + T cells are required for the maintenance of ILC2-induced immunity to N. brasiliensis . ( a ) Number of N. brasiliensis larvae in the lung 2 days post primary infection (Nb), or after intranasal adoptive transfer of CD4 + T cells isolated from naïve mice or mice infected 29 days before transfer ( n =5 mice, mean+s.e.m., representative of two independent experiments, ANOVA). ( b ) Number of N. brasiliensis larvae in the lungs of mice 2 days post primary infection (Nb) and i.v. reinfection (Nb+Nb), or after CD4 + T-cell depletion before primary infection (αCD4+Nb+Nb), and 7 days or 24 h before secondary infection (Nb+αCD4+Nb; n =5 mice, mean+s.e.m., representative of two independent experiments, ANOVA). ( c ) Number of red blood cells in the BALF of mice given a primary (Nb) or secondary (Nb+Nb) infection, and after CD4 + T-cell depletion 7 days before the secondary (Nb+αCD4+Nb). ( d ) Number of ILC2s in the lung of naïve mice or mice 2 days post secondary infection, with or without CD4 + depletion one week before reinfection ( n =3–5, mean+s.e.m., representative of three independent experiments, ANOVA). ( e ) Number of IL-13 + ILC2s in the lung 2 days post challenge infection or with CD4 + depletion one week before reinfection ( n =5, mean+s.e.m., representative of two independent experiments, t -test). ( f ) Mean fluorescent intensity of CD25 expression on lung ILC2s, as in e . ( g ) Differential larvae number in the airways and lung parenchyma of mice with primary (Nb) or i.v. reinfection (Nb+Nb), after CD4 depletion and/or intraperitoneal IL-2C treatment for 7 days before challenge ( n =5, mean+s.e.m., representative of two independent experiments, ANOVA). ( h ) Number of ILC2s in the lungs of i.v.-primary infected (Nb) or reinfected (Nb+Nb) mice, and with CD4 depletion and IL-2C treatment for 7 days before challenge ( n =5, mean+s.e.m., ANOVA). NS, non-significant; P >0.05; ▪ P <0.07; * P <0.05; ** P <0.01; *** P <0.001; **** P <0.0001. Full size image In line with reports by others and our own observations, we hypothesized that CD4 + T cells may have a role in supporting the ILC2 effector population to ensure the maintenance of long-term immunity to reinfection. Interestingly, CD4 depletion at least 1 week before i.v. reinfection with Nb leads to a significant decrease in the number of ILC2s, IL-13 production by ILC2s and the expression of IL-2 receptor by ILC2s ( Fig. 6d–f ). This was in contrast to CD4 depletion of naïve mice before primary i.v. infection where the ILC2 numbers actually increased, most probably reflecting a response of ILC2s to an increase in available niches [20] ( Fig. 6d ). Immunity to reinfection could be restored in these CD4-depleted mice by administration of IL-2C and was also associated with an increase in ILC2 numbers and activation as seen in control reinfected mice ( Fig. 6g,h ). Taken together, these results demonstrate that the ILC2s are required for the protection for naturally acquired lung immunity to Nb, and that ILC2 maintenance is regulated by CD4 + T cells, possibly through IL-2 production [25] , [28] . Lung M2 macrophages mediate Nb killing The increase in macrophage numbers seen in the lungs of i.v.-reinfected mice ( Fig. 7a ), the dependence of immune-mediated worm killing on STAT6 signalling in the lung and the associated IL-4/IL-13 production by CD4 + T cell and ILC2s suggests that alternatively activated M2 macrophages may mediate worm killing in the lung. This is supported by previous studies that have shown that the M2 phenotype within the lung-resident macrophage population is maintained for a significant period of time after Nb infection [10] , [29] , [30] , similar in time frame to the long-lasting immunity to Nb reinfection we observe in our models [7] . To test the involvement of M2 macrophages in lung larvae killing, we derived macrophages from bone marrow of either C57BL/6 or Stat6 −/− donors, cultured in M2 biasing conditions and adoptively transferred these via intranasal administration into the lungs of C57BL/6 naïve mice followed by i.v. infection with Nb. Mice receiving C57BL/6 M2 significantly reduced the numbers of viable worms in the lung to the level seen in i.v.-reinfected mice, whereas mice receiving macrophages from Stat6 −/− donors had no impact on worm viability, suggesting that activation of M2 is sufficient to induce lung immunity to Nb ( Fig. 7b ). 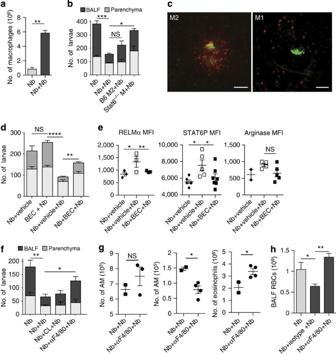Figure 7: M2 macrophages mediate immunity to Nb reinfection. (a) Number of macrophages in the lung in primary (Nb) or i.v.-reinfected mice (Nb+Nb) withN. brasiliensis(n=5, mean+s.e.m., representative of three independent experiments,t-test). (b) Differential larvae number in the airways (dark grey) or lung parenchyma (light grey) of C57BL/6 mice after primary (Nb) or i.v. reinfection (Nb+Nb). Bone marrow-derived M2 from C57BL/6 or Stat6−/−mice were adoptively transferred by intranasal inoculation before infection (n=5 mice, mean+s.e.m., representative of two independent experiments, ANOVA). (c) Confocal imaging of lungs 1 day after i.v. inoculation of CFSE-labelled Nb and 2 days after intranasal transfer with PKH26-labelledbone marrow-derived M2 or M1 macrophages. Images were acquired on live lung tissue, 24 h after infection. Maximum projection of 30zstacks representing an overall 100-μm depth. Scale bar, 100 μm (d) Differential larvae number in the airways or lung parenchyma of mice treated with the arginase inhibitor BEC before primary or i.v. reinfection (n=5 mice, mean+s.e.m., representative of two independent experiments, ANOVA). (e) MFI of RELMa, STAT6P and arginase in interstitial macrophages from mice treated with the arginase inhibitor BEC before i.v.-reinfection infection (n=5 mice, mean+s.e.m., representative of two independent experiments, ANOVA) (f) Differential larvae number in the lungs at day 2 post-primary (Nb) or i.v. reinfection (Nb+Nb), and in mice treated with clodronate liposomes (CL) or anti-F4/80 (Hb-198) antibody or matched isotype control (n=5 mice, representative of two independent experiments, ANOVA). (g) Number of alveolar macrophages (AM, CD45+F4/80intCD11chighSiglecF+), interstitial macrophages (IM, CD45+F4/80highCD11clowSiglecF−) and eosinophils (CD45+F4/80intCD11c−SiglecF+) after i.v. reinfection and with anti-F4/80 administration before reinfection (n=4 mice, mean+s.e.m., representative of two independent experiments, ANOVA). (h) Number of red blood cells in the BALF of mice after primary (Nb) and secondary infection (Nb+Nb) or with anti-F4/80 treatment before i.v. reinfection (Nb+αF4/80+Nb;n=5 mice, mean+s.e.m., ANOVA). NS, non-significant;P>0.05; *P<0.05; **P<0.01; ***P<0.001; ****P<0.0001. Figure 7: M2 macrophages mediate immunity to Nb reinfection. ( a ) Number of macrophages in the lung in primary (Nb) or i.v.-reinfected mice (Nb+Nb) with N. brasiliensis ( n =5, mean+s.e.m., representative of three independent experiments, t -test). ( b ) Differential larvae number in the airways (dark grey) or lung parenchyma (light grey) of C57BL/6 mice after primary (Nb) or i.v. reinfection (Nb+Nb). Bone marrow-derived M2 from C57BL/6 or Stat6 −/− mice were adoptively transferred by intranasal inoculation before infection ( n =5 mice, mean+s.e.m., representative of two independent experiments, ANOVA). ( c ) Confocal imaging of lungs 1 day after i.v. inoculation of CFSE-labelled Nb and 2 days after intranasal transfer with PKH26-labelledbone marrow-derived M2 or M1 macrophages. Images were acquired on live lung tissue, 24 h after infection. Maximum projection of 30 z stacks representing an overall 100-μm depth. Scale bar, 100 μm ( d ) Differential larvae number in the airways or lung parenchyma of mice treated with the arginase inhibitor BEC before primary or i.v. reinfection ( n =5 mice, mean+s.e.m., representative of two independent experiments, ANOVA). ( e ) MFI of RELMa, STAT6P and arginase in interstitial macrophages from mice treated with the arginase inhibitor BEC before i.v.-reinfection infection ( n =5 mice, mean+s.e.m., representative of two independent experiments, ANOVA) ( f ) Differential larvae number in the lungs at day 2 post-primary (Nb) or i.v. reinfection (Nb+Nb), and in mice treated with clodronate liposomes (CL) or anti-F4/80 (Hb-198) antibody or matched isotype control ( n =5 mice, representative of two independent experiments, ANOVA). ( g ) Number of alveolar macrophages (AM, CD45 + F4/80 int CD11c high SiglecF + ), interstitial macrophages (IM, CD45 + F4/80 high CD11c low SiglecF − ) and eosinophils (CD45 + F4/80 int CD11c − SiglecF + ) after i.v. reinfection and with anti-F4/80 administration before reinfection ( n =4 mice, mean+s.e.m., representative of two independent experiments, ANOVA). ( h ) Number of red blood cells in the BALF of mice after primary (Nb) and secondary infection (Nb+Nb) or with anti-F4/80 treatment before i.v. reinfection (Nb+αF4/80+Nb; n =5 mice, mean+s.e.m., ANOVA). NS, non-significant; P >0.05; * P <0.05; ** P <0.01; *** P <0.001; **** P <0.0001. Full size image As M2 macrophages have been shown to be involved in the protective immune response in the gut against H. polygyrus reinfection [31] , we sought to determine whether M2 macrophages could play a similar role in the trapping of Nb in the parenchyma of the lung. We could confirm by fluorescent imaging that M2 macrophages were concentrated in a foci of inflammatory cells that surrounded worms in the parenchyma of reinfected mice, while M1 did not cluster around larvae ( Fig. 7c , Supplementary Movie 1 ). M2 activation markers were reduced in Il-4 −/− and IL-13-depleted mice to the same extent while double depletion of IL-13/IL-4 did further reduce arginase and RELMa expression ( Supplementary Fig. 6a ). M2 are noted for their production of the enzyme arginase and its role in killing parasites [30] , [31] , [32] . Treatment of immune mice reinfected with Nb with the arginase inhibitor S -(2-boronoethyl)- L -cysteine (BEC) partially reversed the killing of worms in the lung airways and the activation phenotype of M2 macrophages ( Fig. 7d,e ) further implicating the M2 macrophages in the trapping and killing of Nb. We depleted alveolar macrophages using clodronate-containing liposomes as previously described [33] , [34] , with two doses of clodronate liposomes being used, including 2 days before infection to ensure macrophage depletion occurs before larvae are introduced ( Supplementary Fig. 6b ), and a second dose at 11 h following infection for maintenance of depletion. Although this treatment regime partially depleted alveolar macrophages, it failed to deplete interstitial macrophages ( Supplementary Fig. 6d–f ), due to the limited capacity of the liposomes to penetrate the phospholipid bilayers as previously shown [33] . Depletion of alveolar macrophages did not affect protection, but the depletion was not sufficient to fully exclude their involvement in protection ( Fig. 7f ). We thus used anti-F4/80 antibody treatment to deplete the interstitial macrophage subset [35] , which lead to a significant decrease in interstitial macrophages but not alveolar macrophages and a decrease in killing of worms ( Fig. 7f,g , Supplementary Fig. 6c–e ) that was associated with the reappearance of haemorrhagic sequalae in the lung ( Fig. 7h ). A role for inflammatory monocytes was ruled out as anti-Gr1 depletion did not affect the loss of worm viability seen in immune mice [36] , [37] ( Fig. 3a ). Taken together, these results prove that at least interstitial M2 macrophages are required for Nb killing in the lung. M2-mediated immunity is sustained by CD4 T + cells and ILC2 M2 macrophages have been shown to be active directly following injury but do require CD4 + T-cell-mediated IL-4/IL-13 expression to sustain their long-term activation [38] . As ILC2s and CD4 + T cells are the main required source of IL-4/IL-13 in the lung during Nb reinfection, we hypothesized that both cell types could play a role in the activation and maintenance of M2 macrophages. This was confirmed with our observation that the Nb-induced increase in lung macrophage numbers was significantly reduced in i.v.-reinfected mice following CD4 + T-cell depletion ( Fig. 8a ), and these macrophages had a reduced expression of both arginase and RELMa ( Fig. 8b ). 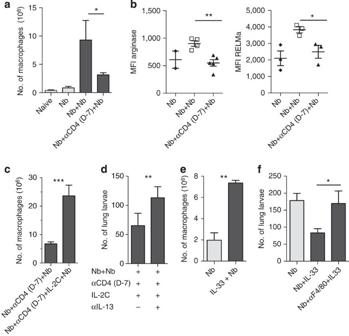Figure 8: Cooperation between ILC2s and T cells allows the long-term maintenance of lung M2 macrophages. (a) Number of macrophages in the lung in naïve, primary (Nb), i.v. reinfection (Nb+Nb) or i.v. reinfection with CD4+T-cell depletion 7 days before the challenge withN. brasiliensis(n=5 mice, mean+s.e.m., representative of two independent experiments, ANOVA). (b) Mean fluorescent intensities of Arginase 1 and RELMα, in the interstitial macrophage population after primary (Nb) and i.v. reinfection (Nb+Nb) and after i.v. reinfection infection with CD4+T-cell depletion 7 days before the reinfection (n=3–5 mice, mean+s.e.m., representative of two independent experiments, ANOVA). (c) Number of macrophages in the lung in i.v. reinfection with CD4+T-cell depletion 7 days before the reinfection with or without IL-2C treatment during the period of CD4 depletion (n=5 mice, mean+s.e.m., representative of two independent experimentst-test). (d) Number of lung larvae in mice i.v. reinfected with Nb with CD4+T-cell depletion 7 days before the reinfection with IL-2C treatment during the period of CD4+depletion and with or without IL-13 blockade during the period of CD4 depletion (n=4 mice, mean+s.e.m.,t-test) (e) Number of macrophages in the lung 2 days post-primary i.v.-infection (Nb), and with anti-CD4 and rmIL-33 or PBS treatment with or without anti-F4/80 treatment or matched isotype control (n=5 mice, mean+s.e.m.,t-test). (f) Number ofN. brasiliensislarvae in the lung 2 days post-primary i.v. infection (Nb) and with anti-CD4 and rmIL-33 or PBS treatment with or without anti-F4/80 treatment or matched isotype control (n=5 mice, mean+s.e.m., ANOVA). *P<0.05; **P<0.01; ***P<0.001. Figure 8: Cooperation between ILC2s and T cells allows the long-term maintenance of lung M2 macrophages. ( a ) Number of macrophages in the lung in naïve, primary (Nb), i.v. reinfection (Nb+Nb) or i.v. reinfection with CD4 + T-cell depletion 7 days before the challenge with N. brasiliensis ( n =5 mice, mean+s.e.m., representative of two independent experiments, ANOVA). ( b ) Mean fluorescent intensities of Arginase 1 and RELMα, in the interstitial macrophage population after primary (Nb) and i.v. reinfection (Nb+Nb) and after i.v. reinfection infection with CD4 + T-cell depletion 7 days before the reinfection ( n =3–5 mice, mean+s.e.m., representative of two independent experiments, ANOVA). ( c ) Number of macrophages in the lung in i.v. reinfection with CD4 + T-cell depletion 7 days before the reinfection with or without IL-2C treatment during the period of CD4 depletion ( n =5 mice, mean+s.e.m., representative of two independent experiments t -test). ( d ) Number of lung larvae in mice i.v. reinfected with Nb with CD4 + T-cell depletion 7 days before the reinfection with IL-2C treatment during the period of CD4 + depletion and with or without IL-13 blockade during the period of CD4 depletion ( n =4 mice, mean+s.e.m., t -test) ( e ) Number of macrophages in the lung 2 days post-primary i.v.-infection (Nb), and with anti-CD4 and rmIL-33 or PBS treatment with or without anti-F4/80 treatment or matched isotype control ( n =5 mice, mean+s.e.m., t -test). ( f ) Number of N. brasiliensis larvae in the lung 2 days post-primary i.v. infection (Nb) and with anti-CD4 and rmIL-33 or PBS treatment with or without anti-F4/80 treatment or matched isotype control ( n =5 mice, mean+s.e.m., ANOVA). * P <0.05; ** P <0.01; *** P <0.001. Full size image To determine whether ILC2s alone could maintain the long-term M2 macrophage population in this Nb infection setting, we used treatment with IL-2C to increase the survival of ILC2s in the absence of T cells, where we observed that macrophage number is no longer restricted by CD4 depletion ( Fig. 8c ). This ILC2-induced effect proved to be dependent on IL-13 as treatment of IL-4-deficient mice with anti-IL-13-neutralizing antibodies in the IL-2C-maintained protection model abrogated the observed increases in macrophage activation and immunity to Nb ( Fig. 8d ). We next investigated the link between ILC2s and M2 macrophages in a model of rmIL-33 induction of ILC2s. Macrophage numbers were increased after IL-33 administration ( Fig. 8e ), and depletion of macrophages by anti-F4/80 administration reversed the protection previously observed on administration of rmIL-33 ( Fig. 8f ). Importantly, the STAT6-dependent nature of the IL-33-induced worm killing excluded that activation by IL-33 worked by the direct activation of macrophages into a M2 phenotype [39] , thus linking ILC2s to a potential role in the activation and maintenance of M2 macrophage function in the lungs following infection with Nb. In this study, we demonstrate the potential of both ILC2 and CD4 + T-cell-mediated regulation of M2-mediated worm killing through the expression of IL-4 and/or IL-13. An intriguing finding was that ILC2s and CD4 + T cells could each act either in concert or directly depending on the activation pathway invoked by worm infection. These included the rapid expansion of IL-13-producing ILC2s in the lung by the alarmin IL-33, leading to a significant reduction in worm survival. Our work thus adds to the previous studies showing that IL-33 is required for lung ILC2s expansion in reinfection and important for the gut expulsion phase of the immune response against Nb with evidence for a role in reducing worm induced damage in the lungs [24] , [27] . Recent papers have demonstrated that ILC2s are important in building a bridge between innate and adaptive immune responses, notably through MHC (major histocompatibility complex) class II interaction and antigen presentation [28] , [40] , [41] . However, in spite of the demonstration that T cells could maintain ILC2s to mediate the expulsion of Nb from the gut 10 days post infection [15] , it remained unclear whether the ILC2s could play a role in an anamnestic response. Here we demonstrate that ILC2s are sufficient and required for macrophage-mediated trapping and killing of Nb in the lungs during the immune response mediating protection against reinfection by Nb. Exogenous administration of IL-2C or IL-33 leading to the activation and increased numbers of IL-13-producing ILC2s promoted worm killing. We propose that IL-33 and IL-2 represent two different regulatory pathways for activating ILC2s and note that TSLP and IL-25, which can also promote ILC expansion, are not required for Nb protection [42] , [43] , suggesting a specialized in vivo role for each of these cytokines [44] , rather than redundant roles. It has been previously shown that the anamnestic protection against Nb is CD4 + T-cell-independent when CD4 depletion occurs 2 days before reinfection [45] while also CD4-dependent as proven by absence of immunity in MHC class II-deficient mice [7] . Our study supports these findings, and provide the explanation for these seemingly contradictory findings. These data provide a more complete view of the role of CD4 + T cells in mediating responses against helminths in the lung with the finding that depletion of CD4 + T cells 7 days before reinfection results in a loss of immunity. The finding that T cells are not required to be present at the moment of challenge, but are required within the preceding week, most likely indicates the importance of T cells for the maintenance of the alternative activation of lung macrophages possibly through the aegis of ILC2-mediated IL-13 production. Our observation that treatment of infected mice with exogenous IL-2C maintains the ILC2 population, in the absence of CD4 + T cells, and maintains the M2 macrophage population in the lung clearly identifies a non-CD4 + T-cell source of IL-13 involved in reducing the viability of the worms in the lung. Given that the number of ILC2s and CD4 + T cells producing IL-13 are equivalent during a secondary infection with Nippostrongylus , it is probable that the two pathways may work in concert to ensure efficient long-term immunity. Recently, Gause and colleagues [18] demonstrated that neutrophils could prime a long-lived effector macrophage population that is important for the rapid expulsion of Nb from the gut during a secondary infection. Ym1 overexpression has recently been shown to result in a swarm of neutrophils around Nb larvae in the lungs, and to damage the worm. However, as Ym1 overexpression also increased the number of alveolar and interstitial macrophages, it is possible that neutrophils/macrophages cooperate to drive Nb killing in the lung [46] . While we certainly agree on the sufficiency of the M2 phenotype of macrophages for immune killing of Nb [18] , we have not been able to demonstrate any role for neutrophils in this mechanism in the lung. Given that the neutrophils are recruited faster than CD4 + T cells or ILC2s after Nb infection, they may be important in the initial priming of the macrophages, while CD4 + T cells and ILC2s could participate in the long-term maintenance of the M2 phenotype. Moreover, our study strengthens the role of M2 macrophages in the anamnestic response against Nb by demonstrating the specific requirement of interstitial macrophages for protection in the lung. In light of our findings that support the same type-2 effector mechanisms being involved in lung repair after Nb-induced damage and in protection, it is interesting to note that Turner et al. [13] recently reported that Il-9r −/− mice, that are unable to repair lung damage after Nb infection due to a deficiency in ILC2s, show an associated reduction in M2 markers of interstitial but not alveolar macrophages. Our results place the lungs as an important component of the type-2 immune response against helminths that confers resistance to reinfection. Several important parasites of man and animals have evolved a common infection strategy involving migration through the lungs. Improved understanding of the immunological mechanisms underpinning the lung response holds the promise for therapeutic approaches to establish immunity against these ancient pathogens. Mice Wild-type mice or mice with either Stat6 −/− (The Jackson Laboratory), G4/G4 (ref. 47 ) (Il-4 −/− ), 4C13R [20] or Rag1 −/− (The Jackson Laboratory), gene modifications, all on a C57Bl/6J background or Il-3 −/− (Cleveland Clinic, USA) on a BALB/c background, were bred by the Biomedical Research Unit, Malaghan Institute of Medical Research, Wellington, New Zealand. Mice were used at 6–10 weeks of age and sex matched. All experimental procedures used were approved and carried out as approved by the Victoria University of Wellington, Wellington, New Zealand. Preparation and isolation of N. brasiliensis larvae Nb is maintained by monthly passage in Lewis rats. Infective (iL3) worms were prepared from 2-week rat fecal cultures as originally described [48] . Larvae migrating to the lung (2 h after i.v. administration, 18 h after s.c. or 48 h after i.v. when stated in the legend) were harvested by digestion of diced lung tissue in IMDM, 0.1 mg ml −1 of liberase TL (Roche), 120 μg ml −1 DNAse I (Roche) at 37 °C with agitation for 45 min. Larvae were separated from the tissue homogenate by sequential filtration through 100-μm cell strainer and 40-μm cell strainers. Viable larvae were recovered from tissue (lung or gut) by dicing wrapping in cheesecloth to form a bag and suspending at the surface of a 50-ml centrifuge tube containing PBS at 37 °C for at least 2 h. Viable worms follow a thermal gradient and migrate out of the bag to collect at the bottom for counting [48] . Larvae present in the large airways were harvested by bronchoalveolar lavage, with 3 × 1 ml of PBS. Infection with Nb was initiated by either s.c. or i.v. routes with 550 live iL3 in 200 or 50 μl of sterile PBS respectively. D0 marks the day of infection. If not explicitly mentioned, the time between primary and reinfection was 30 days. The protection percentage is calculated as (1−number of worms in reinfected mouse/average number of worms in primary infected mice) × 100. Six hundred dead larvae or polystyrene beads (30 μm diameter, Sigma-Aldrich) were injected i.v. as controls for the airways migration experiment. Injected worms were fluorescently labelled to track their distribution in the skin following infection, and the skin area containing worms was harvested and then submitted to gastric juice digestion, as described previously [5] . Preparation of bone marrow-derived macrophages Bone marrow-derived macrophages were generated by 7-day culture of bone marrow cells with supernatant from a macrophage colony-stimulating factor-secreting cell line (L929, Otago University, Dr Alex McLellen) as previously described [49] . On day 7 of culture, Bone marrow-derived macrophages were either left untreated, exposed to recombinant IL-4 (CHO mIL-4, Basel, 10 U ml −1 ) for 24 h or interferon-γ (Peprotech, 100 U ml −1 ) for 12 h. The activation and purity of the specific macrophage subsets was confirmed by flow cytometry before adoptive transfer or worm co-culture. For adoptive transfer, 1.7 million cells were administered intranasally in 50 μl of PBS, following PKH26 labelling (Sigma-Aldrich) labelling according to the manufacturer’s instructions. In vivo treatment IL-33 (50 μl) or control PBS (10 μg ml −1 ) were administered intranasally. IL-2C or control PBS were administered intraperitoneally as previously reported [20] (IL-2, Peprotech, aIL-2, clone JES6-1A12 BioXcell). Lung macrophage depletion was as previously described [33] ; briefly, clodronate- or PBS-liposomes solution (50 μl) was administered intranasally 48 h before and 11 h after the initiation of reinfection with Nb. For intranasal administration of cytokines or liposomes, mice were lightly anaesthetized with xylazine and ketamine for the duration of the inoculation procedure. The arginase inhibitor (BEC) was administered in the drinking water supplemented with sweetener (0.25 % BEC, sweetener (Splenda) 4 g l −1 ) for 24 h, 1 day before infection with Nb. Antibodies anti-F4/80 (ref. 35 ); HB-198 hybridoma; ATCC, 0.250 mg), anti-CD4 (GK1.5, BioXcell, 0.5 mg), anti-CD90 (30H12, BioXcell, 0.5 mg), anti-Gr1 (ref. 36 ; RB6–8C5, 0.250 mg) anti-IL-13 (generously provided by AbbVie, 1 mg) were administered intraperitoneally. Anti-F4/80 antibodies were administered 2 days before challenge and 1 day after challenge. For ILC2s depletion, anti-CD90 was administered every day from the fourth day before the i.v. administration of larvae, and 1 day after infection. IL-2C was given 2 days before infection. IL-13 was blocked for a week before reinfection, with two administrations of anti-IL-13. For T-cell depletion, anti-CD4 was administered 7 days and 3 days before challenge or 1 day before challenge. IL-2C was administered every 2 days from day −7. Isolation of lung tissue and BALF Lung tissue was minced with scissors, followed by digestion in DMEM medium containing Collagenase type I (2.4 mg ml −1 , Sigma-Aldrich, St Louis, MO) and DNase I (120 μg ml −1 ; Sigma-Aldrich, St Louis, MO) for 1 h at 37 °C with agitation. Samples were further disassociated by repeated passage through a 5-ml syringe fitted with an 18-gauge needle and finally passed through a 100-μm cell strainer to obtain a single-cell suspension. BALF was collected using established protocols. For cytokine analysis, the first ml of wash was used. For larvae count and red blood cell count, the 3-ml of wash were pooled together. Larvae were manually counted under bright field on a stereomicroscope. Red blood cells were counted with a haemocytometer, after centrifugation of the BALF and resuspended in 1 ml to account for the difference of BALF volume harvested in each mouse. Flow cytometric analysis Isolated cells were resuspended in FACS buffer, and Fc-receptors were blocked (2.4G2) before staining with monoclonal antibodies before collection on a Fortessa flow cytometer (BD) or LSRII flow cytometer (BD). Fluorochrome-conjugated antibodies to the following cell surface molecules were used: CD3-PE-Cy7 (2C11, eBiosciences), CD4-FITC (RM4-4, BD Biosciences Pharmingen), CD8-AF700 (53–6.7, Biolegend), CD44-APC (IM7, BD Biosciences Pharmingen), CD62L-Biotin (MEL-14, BD Biosciences Pharmingen), CD45-APC-Cy7 (30-F11, BD Biosciences Pharmingen), NK1.1-PerCP-Cy5.5 (PK136, BD Biosciences Pharmingen) for T-cell analysis; CD90-Brilliant Violet (53–2.1, Biolegend), CD90-APC (53–2.1, BD Biosciences Pharmingen), CD25-FITC (7D4, BD Biosciences Pharmingen), CD25-PE (PC61, BD Biosciences Pharmingen), CD2-Biotin (RM2–5, BD Biosciences Pharmingen), CD3-PerCP-Cy5.5 (145–2C11, BD Biosciences Pharmingen), CD11b-PerCP-Cy5.5 (M1/70, BD Biosciences Pharmingen), CD45-APC-Cy7 (30-F11, BD Biosciences Pharmingen), B220-PE-CF594 (RA3–6B2, BD Biosciences Pharmingen), NK1.1-PerCP-Cy5.5 (PK136, BD Biosciences Pharmingen), ST2-FITC (DJ8, MD Bioproducts), GATA3-AF647 (L50–823, BD Biosciences Pharmingen) for ILC2s; CD90-BV605 (53–2.1, Biolegend), CD200R3-APC (Ba13, Biolegend), CD45-APC-Cy7 (30-F11, BD Biosciences Pharmingen) for basophils; CD45-PerCpCy5.5 (30-F11, BD Biosciences Pharmingen), F4/80-APCeF780 (BM8, Ebiosciences), CD11c-APC (HL3, BD Biosciences Pharmingen), RELMa-PECy7 (226033, R&D systems), STAT6P-PE (PY641, BD Biosciences Pharmingen), Arginase-PECy7 (Abcam), SiglecF-PE (E50–2440, BD Biosciences Pharmingen) for macrophages and eosinophils. Cell suspensions were resuspended in running buffer containing 0.5 μg ml −1 DAPI (4′,6-diamidino-2- phenylindole dihydrochloride; Molecular Probes, Invitrogen) for the exclusion of dead cells or stained with LIVE/DEAD fixable blue dead cell Stain kit (Invitrogen) when fixation was required for intracellular staining. Analysis was performed with the FlowJo software (Treestar). ILC2s were identified most of the time as CD45 + Lineage − CD90 + CD25 + . In the experiments where ILC2s were depleted with aCD90, ILC2s were identified as CD45 + Lineage − CD25 + Gata3 + , as we found masking of CD90 following the antibody-depletion treatment. Alveolar macrophages were identified as CD45 + F4/80 int CD11c high SiglecF + , interstitial macrophages as CD45 + F4/80 high CD11c low SiglecF − and eosinophils as CD45 + F4/80 int CD11c − SiglecF + . Dye labelling of live parasites For external labelling (that is, the sheath), iL3 were washed several times in PBS, incubated at room temperature for 8 min in 2.5 mM carboxyl fluorescein succinimidyl ester (CFSE, Sigma-Aldrich) and then washed in PBS three times before infection of the host. For internal labelling, iL3 were sterilized by washing in antibiotics and then fed with Fluorosbrite YO carboxylate microsphere (Polysciences Inc.) beads for 4 h. The larvae were then washed in PBS, 0.05 % Tween before infection of the host. The efficiency of staining and viability iL3 was verified by microscopy before infection. Fluorescent imaging of larvae in lungs and analysis C57BL/6 mice were injected i.v. with double-labelled L3. Mice were euthanized 5 min or 8 h after infection, and the lungs were removed for imaging. Dispersion of the larvae was recorded with a SZX 16 fluorescent stereomicroscope (Olympus, Japan). Adoptively transferred macrophages were labelled with PKH26 following the manufacturer’s instructions and washed three times in PBS, 10% bovine serum albumin before intranasal administration. Fluorescent larvae were inoculated the next day. Immediately after euthanasia, the lungs were placed in a six-well plate in PBS, and placed in a dark box until observation. Fluorescence was recorded with a FV 1200 confocal microscope (Olympus, Japan). Samples were imaged through a × 20 objective. For detection of fluorophores, samples were exposed to diode laser light at a wavelength of 473 nm for the excitation of both PKH26 and CFSE, and the fluorescence was detected through 515/50 and 680/100 filters respectively. Image stacks were transformed into movies or maximum projection with ImageJ [50] . Larvae morphology and viability The following parasite features were analysed by light microscopy on materials (fixed in toto with 4% formaldehyde in cold PBS to avoid body shrinkage): (i) size of the larvae, (ii) size of the oesophagus and (iii) molt3. For pigment quantification, larvae were observed live, as fixation destroyed the pigment. Larvae harvested from lungs were cytospun before Giemsa staining to observe potential cell adherence. Larvae were recovered from lungs by a chemotaxis assay and washed thoroughly with PBS to remove all adherent cells, counted and homogenized by a pool of 20 L3s in a bead beater in 100 μl of PBS with 1.1 mm Tungsten carbide beads (BioSpec Products Inc.). ATP levels in larval homogenates were analysed by CellTiter-Glo Luminescent Cell Viability Assay [31] (Promega, Madison, WI). Preparation of clodronate liposomes Liposomes were prepared from stock solutions of phosphatidyl choline (100 mg ml −1 in CHCl 3 , Sigma-Aldrich), cholesterol (10 mg ml −1 in CHCl 3 , Sigma-Aldrich) and sodium clodronate based on the method of van Rooijen [33] . Preparation of BEC BEC was synthesized as described by Matteson [51] , [52] , except that vinylmagnesium bromide was used in the reaction with trimethylborate for the first step of the synthesis [53] . Lung histopathology Lung tissues were harvested from naïve and Nb-infected mice into 10% formalin before embedding in paraffin. Sections (10-μm thin) were cut and stained by the standard haematoxylin and eosin procedure. Statistical analysis The choice of statistical tests was based on sample size and on Bartlett’s test when normal distributions of the errors were expected. Data from separate experiments were pooled when possible. Total lung or skin numbers were analysed by ANOVA (analysis of variance, one or two way) or by t -test when only two groups were compared, while distribution in the parenchyma or in the BALF was analysed using a logistic regression model (odds ratios are presented in Supplementary Fig. 6 ). Morphology parameters were analysed using t -tests. Data were excluded only based on error of manipulation (incomplete worm injection) or in the case of IL depletion if the treatment did not work, as measured by the number of ILCs. Cell numbers were analysed by t -test or ANOVA. Representation and data analysis were performed with R or GraphPad Prism 5. Statistically significant values are indicated as follows: NS, P >0.05; ▪ P <0.07; * P <0.05; ** P <0.01; *** P <0.001; **** P <0.0001. How to cite this article: Bouchery, T. et al. ILC2s and T cells cooperate to ensure maintenance of M2 macrophages for lung immunity against hookworms. Nat. Commun. 6:6970 doi: 10.1038/ncomms7970 (2015).